Large-scale mutational analysis of Kv11.1 reveals molecular insights into type 2 long QT syndrome It has been suggested that deficient protein trafficking to the cell membrane is the dominant mechanism associated with type 2 Long QT syndrome (LQT2) caused by Kv11.1 potassium channel missense mutations, and that for many mutations the trafficking defect can be corrected pharmacologically. However, this inference was based on expression of a small number of Kv11.1 mutations. We performed a comprehensive analysis of 167 LQT2-linked missense mutations in four Kv11.1 structural domains and found that deficient protein trafficking is the dominant mechanism for all domains except for the distal carboxy-terminus. Also, most pore mutations—in contrast to intracellular domain mutations—were found to have severe dominant-negative effects when co-expressed with wild-type subunits. Finally, pharmacological correction of the trafficking defect in homomeric mutant channels was possible for mutations within all structural domains. However, pharmacological correction is dramatically improved for pore mutants when co-expressed with wild-type subunits to form heteromeric channels. Kv11.1 is a voltage-gated K + channel encoded by the human ether-a-go-go-related gene ( hERG or KCNH2 ) and is associated with the pathophysiology of inherited cardiac arrhythmia diseases, including type 2 long QT syndrome (LQT2) [1] , sudden infant death syndrome (SIDS) [2] and short QT syndrome [3] , as well as various forms of cancer [4] , epilepsy [5] and schizophrenia [6] . Nearly 500 KCNH2 mutations have been linked to LQT2—which is characterized by a prolonged time duration from ventricular depolarization to repolarization (QT interval on an ECG)—and increased risk for sudden cardiac death. These loss-of-function mutations have been classified into four molecular mechanisms: class 1, abnormal transcription/translation; class 2, deficient protein trafficking; class 3, abnormal channel gating/kinetics; and class 4, altered channel permeability, in all of which the repolarizing outward K + current, I Kv11.1 or I Kr , is reduced [7] . While a fraction of KCNH2 mutations are nonsense and are postulated to invoke a class 1 mechanism due to nonsense-mediated mRNA decay [8] , the majority are missense mutations, with most postulated to invoke a class 2 mechanism due to protein misfolding and endoplasmic reticulum-associated degradation (ERAD) [9] , [10] , [11] , [12] . Interestingly, for some trafficking-deficient mutations, the defect can be corrected pharmacologically (usually with high-affinity Kv11.1 channel blockers), with reduced culture temperature, or by RNA interference [10] , [13] , [14] , [15] , [16] , suggesting therapeutic potential for LQT2 carriers, although application of these findings to LQT2 patients remains a major challenge. In addition, of the >300 missense mutations, most remain functionally uncharacterized and are spread throughout the Kv11.1 multidomain protein, which contains voltage sensor (VSD, S1–4) and pore (S5–6) domains comprising the transmembrane domain (TMD) [17] , an amino-terminus containing the PerArntSim domain (PASD) with PAS-cap collectively making up a conserved ‘EAG’ domain present in the EAG family of Kv channels [18] , and a carboxy-terminus containing the cyclic-nucleotide-binding homology domain (CNBHD) [19] along with a distal C-terminal ER retention signal (RXR) [20] and coiled-coil domain (CCD) [21] . Furthermore, carriers of LQT2 mutations are heterozygous, making co-assembly dynamics (dominant negative, haploinsufficiency) of the tetrameric channel another factor contributing to disease complexity [22] . While much has been learned about the molecular basis underlying LQT2 (ref. 23 ), many important gaps remain, three of which we address in this paper. 1 Not all mutations characterized in heterologous expression systems show a loss-of-function phenotype, suggesting that some reported mutations may be benign sequence variants or single-nucleotide polymorphisms (SNPs) [10] , [24] . This emphasizes the need to functionally express and analyse individual mutations. 2 The location of a mutation within the Kv11.1 protein may be important, but the molecular basis for this is unknown. Mutations in the pore clinically have a more severe phenotype [25] , [26] . Several lines of evidence suggest that TMD (including pore) and CNBHD mutations invoke a class 2 (trafficking-deficient) mechanism [10] , [27] versus intracellular (‘core’) mutations that may traffic normally and exert a class 3 (abnormal gating) mechanism [28] . ‘Core’ interactions between the PASD, S4–S5 linker and CNBHD regulate Kv11.1 gating [29] , [30] , [31] , [32] , [33] , [34] , [35] , and many engineered and LQT2-linked ‘core’ mutations exhibit more rapid deactivation [18] , [32] , [36] . A recent study reported that some PASD mutations traffic normally [28] . Alternatively, differences may be attributed to differences in wild type (WT)–mutant subunit interactions. Several intracellular mutations reduce I Kv11.1 in a partially dominant-negative manner or through haploinsufficiency [10] , [37] , [38] , [39] , while most pore mutations have a strong dominant-negative interaction with WT subunits producing little to no current [10] , [14] , [40] , [41] . Unfortunately, most LQT2 mutations remain functionally uncharacterized and the disease mechanisms are unknown. 3 Studies using mostly homomeric channels show that culture in the presence of pore-blocking drugs such as E4031, which involve π-cation, π–π stacking and hydrophobic interactions with aromatic residues in TMD S6 (refs 42 , 43 ), can correct defective protein trafficking of some mutations in the TMD (pore and VSD) and PASD [10] , [38] , [44] . Second-site S6 mutations can also correct some pore mutations [45] . These findings and the observation that E4031-corrected channels are more resistant to proteases suggest that E4031 correction works by stabilizing the pore, which can also facilitate cooperative folding between domains/subunits, resulting in more tightly packed channels that evade ERAD [46] . However, E4031 correction seems limited primarily to pore domain mutations, along with a few in the PASD and none in the CNBHD [10] , [28] . E4031-dependent pharmacological correction has been studied for relatively few homomeric and even fewer heteromerically (with WT) expressed mutations; thus, a comprehensive analysis of mutations co-expressed with WT subunits across multiple structural domains is needed to better understand pharmacological correction as a potential therapy. In the present work, we undertook a large-scale analysis of LQT2 missense mutations in different structural domains of the Kv11.1 protein to generate new insights about LQT2 disease mechanisms. We studied missense mutations because they are the most commonly identified genetic abnormality in patients with LQT2. We adopted a data-driven approach employing heterologous mammalian expression to generate immunoblot and electrophysiology data, combined with computational structural models, to characterize both homotetrameric (mutant or WT) and heterotetrameric (mutant+WT) channels. We generated and studied 167 LQT2 mutations as well as three KCNH2 SIDS mutations and two SNPs. We showed that 88% of LQT2 missense mutations in the PASD, C-linker/CNBHD and pore domains invoke a class 2 (trafficking-deficient) mechanism, but with some major differences. Over 70% of LQT2 pore mutations were strictly dominant negative, whereas PASD or C-linker/CNBHD mutations were not. In addition, LQT2 mutations in all domains were pharmacologically (E4031) correctable (PASD>pore>C-linker/CNBHD), and this improved dramatically when mutations were co-expressed with WT subunits (pore>PASD>C-linker/CNBHD), making pharmacological correction much more common than previously thought. We also mapped each mutation to structural models to analyse structure/(dys)function relationships. We then combined these results with previously published studies (see supplementary tables ) and discuss here a simplified model for the different Kv11.1 trafficking phenotypes. To our knowledge, this is the largest mutational study for any congenital disease, which should serve as a valuable resource and help spark further inquiry into this ion channelopathy. Trafficking phenotype of homomeric EAGD mutations We compiled a list of 291 LQT2 and 10 SIDS-linked KCNH2 mutations, as well as 28 SNPs (see Methods, Fig. 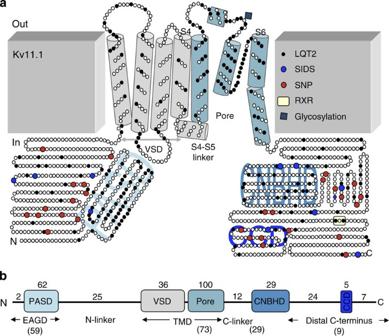Figure 1: Topology of Kv11.1. (a) Cartoon of Kv11.1 with circles representing amino acids and cylinders representing TMD segments 1–6 and the S4–S5 linker. S1–S4 make up the VSD and the pore is located between S5 and S6. The intracellular PASD, CNBHD and CCD are labelled in light blue. Black and blue circles show the location of all reported LQT2 and SIDS mutations, respectively. Red circles show the location of all reported SNPs. The ER retention signal RXR is highlighted in yellow and the glycosylation site at N598 is shown with a blue diamond. (b) Linear representation of the different Kv11.1 domains (to scale) showing the number and domain location of all LQT2-linked and SIDS mutations identified to date. The numbers characterized in this study are in parentheses (59 of 64 mutations for the EAGD, 73 of 100 mutations for the pore, 29 of 41 mutations for the C-linker and CNBHD, and 9 of 36 mutations for the distal C-terminus). 1 and Supplementary Table 1 ). While the TMD contains 1/2 of the LQT2 missense mutations, the PASD is another ‘hotspot’ with at least 62 (61 LQT2, 1 SIDS) mostly uncharacterized mutations at 47 sites. Two more are located in the N-terminal proximal to the PASD in the PAS-cap amphipathic helix (amino acids 13–23) ( Fig. 2c ) [47] . To determine their trafficking phenotype, immunoblot was performed on transiently transfected HEK293 cells expressing homomeric Kv11.1 channels cultured at physiological temperature (37 °C) as well as reduced culture temperature (27 °C for 24 h), or with 10 μM E4031 in the culture medium (24 h) to test for correction. Kv11.1 protein (132 kDa) is synthesized in the ER, where it undergoes N-linked core-glycosylation (135 kDa) and then traffics to the golgi for N-linked complex glycosylation (155 kDa) before reaching the plasma membrane. A doublet on immunoblot (135- and 155-kDa bands) indicates cell surface trafficking, whereas a lack or decrease of the 155-kDa band indicates deficient trafficking [9] , [10] . 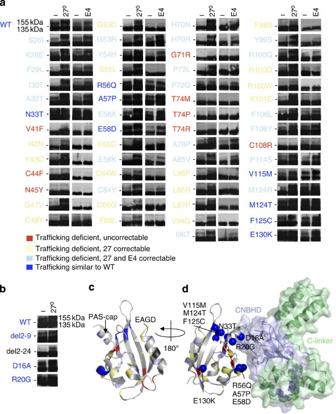Figure 2: Trafficking phenotype and structural context of LQT2-linked EAGD missense mutations. (a,b) Representative immunoblots of transiently transfected HEK293 cells comparing trafficking under control culture conditions at 37 °C, at reduced temperature (27 °C, 24 h) or in E4031 (E4, 24 h). Dashes (−) indicate the 140-kDa molecular weight marker. Mutations are colour-coded as follows: trafficking deficient and uncorrectable in red, trafficking deficient but correctable at 27 °C in yellow, trafficking deficient but correctable at 27 °C or with E4031 in light blue, and those that traffic similar to WT in blue. (c) Crystal structure of the EAGD (PDB: 4HP9). Mapped LQT2 residues correspond to panelaand uncharacterized mutations (I96V and D102A) are in black. (d) Representation of the EAGD (PDB: 4HP9) complexed with the C-linker/CNBHD model from alignments to the structure of the EAGD–CNBHD complex from mouse (PDB: 4LLO). C-linker region is shown in green, CNBHD in blue and intrinsic ligand in magenta. Mutations that are trafficking competent (blue balls) are labelled. An example of a full-length immunoblot can be found inSupplementary Fig. 2. Figure 2a shows representative immunoblots ( n ≧ 2) for 57 PASD mutations, which exhibited four different trafficking phenotypes: trafficking deficient and uncorrectable (red), trafficking deficient but correctable with culture at 27 °C (yellow), trafficking deficient but correctable with culture at 27 °C or with E4031 (light blue), or normal trafficking (blue). Of the 57 mutations, 49 (86%) lacked or had a diminished 155-kDa band on immunoblot compared to WT under control conditions. Among these 40 (82%) were temperature correctable and 23 (47%) were E4031 correctable. Interestingly, 17 were only temperature correctable but none were only E4031 correctable. So, in contrast to a previous study [28] , most PASD mutations are trafficking deficient and correctable. These data, combined with several mutations already reported in the literature, are summarized in Supplementary Table 2 . Figure 1: Topology of Kv11.1. ( a ) Cartoon of Kv11.1 with circles representing amino acids and cylinders representing TMD segments 1–6 and the S4–S5 linker. S1–S4 make up the VSD and the pore is located between S5 and S6. The intracellular PASD, CNBHD and CCD are labelled in light blue. Black and blue circles show the location of all reported LQT2 and SIDS mutations, respectively. Red circles show the location of all reported SNPs. The ER retention signal RXR is highlighted in yellow and the glycosylation site at N598 is shown with a blue diamond. ( b ) Linear representation of the different Kv11.1 domains (to scale) showing the number and domain location of all LQT2-linked and SIDS mutations identified to date. The numbers characterized in this study are in parentheses (59 of 64 mutations for the EAGD, 73 of 100 mutations for the pore, 29 of 41 mutations for the C-linker and CNBHD, and 9 of 36 mutations for the distal C-terminus). Full size image Figure 2: Trafficking phenotype and structural context of LQT2-linked EAGD missense mutations. ( a , b ) Representative immunoblots of transiently transfected HEK293 cells comparing trafficking under control culture conditions at 37 °C, at reduced temperature (27 °C, 24 h) or in E4031 (E4, 24 h). Dashes (−) indicate the 140-kDa molecular weight marker. Mutations are colour-coded as follows: trafficking deficient and uncorrectable in red, trafficking deficient but correctable at 27 °C in yellow, trafficking deficient but correctable at 27 °C or with E4031 in light blue, and those that traffic similar to WT in blue. ( c ) Crystal structure of the EAGD (PDB: 4HP9). Mapped LQT2 residues correspond to panel a and uncharacterized mutations (I96V and D102A) are in black. ( d ) Representation of the EAGD (PDB: 4HP9) complexed with the C-linker/CNBHD model from alignments to the structure of the EAGD–CNBHD complex from mouse (PDB: 4LLO). C-linker region is shown in green, CNBHD in blue and intrinsic ligand in magenta. Mutations that are trafficking competent (blue balls) are labelled. An example of a full-length immunoblot can be found in Supplementary Fig. 2 . Full size image Quickened deactivation from N-terminus truncated channels and LQT2 mutations can be restored by adding back the EAG domain or just the first 16 residues of the PAS cap [18] , [31] , [48] . Binding of the PASD to the CNBHD is thought to position the amphipathic helix and in turn the N-terminal residues near the bottom of S6 to modulate Kv11.1 gating [30] , [34] , [35] . We further tested to see if the PAS cap is also important for trafficking, and found that deletion of residues 2–9 had no effect on trafficking, but that deletion of residues 2–24 containing the amphipathic helix did impair trafficking. The LQT2 mutations D16A and R20G were both trafficking-competent ( Fig. 2b ). Structural and functional properties of EAGD mutations EAGD mutations were mapped onto its structure (PDB: 4HP9) [49] , which has a fold consisting of a central antiparallel β-sheet flanked by several α-helices ( Fig. 2c ). While the different trafficking-deficient phenotypes are scattered, showing no correlation with location, most trafficking-competent mutations lie near its hydrophobic surface, which interfaces with the CNBHD (PDB: 4LLO) [35] , a region important for regulating Kv11.1 deactivation [18] , [50] , [51] ( Fig. 2d ; Supplementary Fig. 1a,b,g,h ). To determine their electrophysiological properties, stably transfected cells were generated for the trafficking-competent D16A, R20G, E58D, V115M, F125C, E130K mutations, as well the trafficking-deficient M124R located near the hydrophobic surface. Representative western blots and peak tail I Kv11.1 densities are shown in Supplementary Fig. 2a . The greatest change in V 1/2 was for D16A and E130K, which were shifted +13 and −10 mV, respectively ( Fig. 3a,b ). Deactivation measured at −50 mV was slower for D16A and faster for M124R compared to WT, consistent with previous reports ( Fig. 3c ) [47] , [52] , and D16A, R20G and E58D all exhibited slightly slower inactivation at 0 mV ( Fig. 3d ). In contrast, the functional properties of E58D, V115M and F125C were similar to WT, suggesting that they may be benign variants ( Table 1 ; Fig. 3a–d ). In addition to M124R, stable cell lines of F106L also exhibited the same trafficking phenotype as transient transfections, showing a weak 155-kDa band on immunoblot, which increased with culture at reduced temperature or with E4031 ( Supplementary Fig. 2d ). 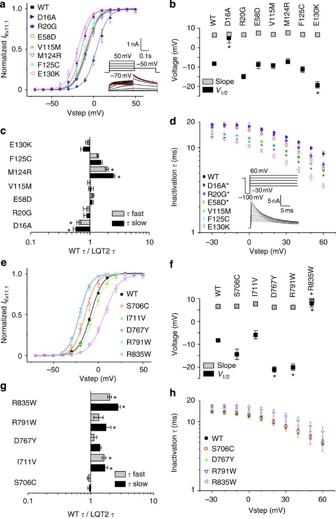Figure 3: Electrophysiological properties of LQT2-linked EAGD and C-linker/CNBHD missense mutations. (a,e) Activation current–voltage (I–V) relationships. From a holding potential of −80 mV, cells were depolarized to voltages between −70 and 50 mV in 10-mV increments for 3 s to quantify the tail current.I–Vrelations were determined by normalizing peak tail currents (Itail) from each step to the maximal peakItail. (b,f)V1/2and slope factors. The voltage at which peakIKv11.1was half-maximal (V1/2) and the slope factor (k) were determined by fitting the normalizedI–Vrelationship with the Boltzmann function. (c,g) WT-to-mutant time constant ratios (speeding factor) for deactivation at −50 mV. The fast (τfast) and slow (τslow) time constants of channel deactivation were determined with a double exponential fit of theItaildecay from 50 to −50 mV (red trace). (d,h) Inactivation time constants determined at 0 mV. From a holding potential of −80 mV, cells were depolarized to 50 mV for 1.5 s to open and inactivate channels, followed by a short 10-ms step to −100 mV to remove inactivation without allowing enough time for the channels to deactivate. This was followed by test pulses from −30 to 60 mV in 10-mV increments. Inactivation time constants for each step were fit with a single exponential. Error bars are s.e.m. Asterisks indicate statistical significance (P≪0.05).n=3 to 9 HEK293 cells for each experiment. Figure 3: Electrophysiological properties of LQT2-linked EAGD and C-linker/CNBHD missense mutations. ( a , e ) Activation current–voltage ( I – V ) relationships. From a holding potential of −80 mV, cells were depolarized to voltages between −70 and 50 mV in 10-mV increments for 3 s to quantify the tail current. I – V relations were determined by normalizing peak tail currents ( I tail ) from each step to the maximal peak I tail . ( b , f ) V 1/2 and slope factors. The voltage at which peak I Kv11.1 was half-maximal ( V 1/2 ) and the slope factor (k) were determined by fitting the normalized I – V relationship with the Boltzmann function. ( c , g ) WT-to-mutant time constant ratios (speeding factor) for deactivation at −50 mV. The fast ( τ fast ) and slow ( τ slow ) time constants of channel deactivation were determined with a double exponential fit of the I tail decay from 50 to −50 mV (red trace). ( d , h ) Inactivation time constants determined at 0 mV. From a holding potential of −80 mV, cells were depolarized to 50 mV for 1.5 s to open and inactivate channels, followed by a short 10-ms step to −100 mV to remove inactivation without allowing enough time for the channels to deactivate. This was followed by test pulses from −30 to 60 mV in 10-mV increments. Inactivation time constants for each step were fit with a single exponential. Error bars are s.e.m. Asterisks indicate statistical significance ( P ≪ 0.05). n =3 to 9 HEK293 cells for each experiment. Full size image Table 1 Electrophysiological properties of Kv11.1 missense mutations. Full size table Trafficking of homomeric CNBHD mutations The C-terminus of Kv11.1 contains a CNBHD coupled to the pore through a C-linker region (C-linker/CNBHD, PDB: 3UKN) [19] . This domain contains at least 41 (39 LQT2, 2 SIDS) mostly uncharacterized mutations at 33 sites. To determine their trafficking phenotype we used the same immunoblot assay and colour-code presentation as described for EAGD. 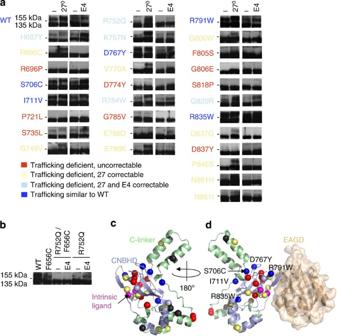Figure 4: Trafficking phenotype and structural context of LQT2-linked C-linker/CNBHD LQT2 missense mutations. (a,b) Representative immunoblots of transiently transfected HEK293 cells comparing trafficking under control conditions at 37 °C, at reduced temperature (27 °C, 24 h) or in E4031 (E4, 24 h). Dashes (−) indicate the 140-kDa molecular weight marker. Mutations are colour-coded as follows: trafficking deficient and uncorrectable in red, trafficking deficient but correctable at 27 °C in yellow, trafficking deficient but correctable at 27 °C or with E4031 in light blue, and those that traffic similar to WT in blue. (c) Model of the C-linker/CNBHD with C-linker region in green, CNBHD in blue and intrinsic ligand in magenta. Mapped LQT2 residues correspond to panelaand uncharacterized mutations (L678P, L693P, I728F) are in black. (d) Representation of the EAGD (coloured wheat) (PDB: 4HP9) complexed with the C-linker/CNBHD model from alignments to the structure of the EAGD–CNBHD complex from mouse (PDB: 4LLO). Figure 4a shows representative immunoblots ( n ≧ 2) for 29 mutations. In all 24(82%) lacked or had a diminished 155-kDa band on immunoblot compared to WT for control (37 °C) culture conditions. Of these, 15 (62%) were correctable with culture at 27 °C and 5 (17%) were correctable with culture in E4031. Similar to the EAGD, 10 mutations were only temperature correctable but no mutations were only E4031 correctable. These data, combined with several mutations already reported in the literature, are summarized in Supplementary Table 3 . Since this is the first report of an E4031 correctable C-terminal mutation, we tested to see if it acts through the same pore drug-binding site [42] , [43] . Indeed, F656C, which traffics normally but attenuates E4031 drug block of I Kv11.1 , abolished E4031 correction of R752Q ( Fig. 4b ). Figure 4: Trafficking phenotype and structural context of LQT2-linked C-linker/CNBHD LQT2 missense mutations. ( a , b ) Representative immunoblots of transiently transfected HEK293 cells comparing trafficking under control conditions at 37 °C, at reduced temperature (27 °C, 24 h) or in E4031 (E4, 24 h). Dashes (−) indicate the 140-kDa molecular weight marker. Mutations are colour-coded as follows: trafficking deficient and uncorrectable in red, trafficking deficient but correctable at 27 °C in yellow, trafficking deficient but correctable at 27 °C or with E4031 in light blue, and those that traffic similar to WT in blue. ( c ) Model of the C-linker/CNBHD with C-linker region in green, CNBHD in blue and intrinsic ligand in magenta. Mapped LQT2 residues correspond to panel a and uncharacterized mutations (L678P, L693P, I728F) are in black. ( d ) Representation of the EAGD (coloured wheat) (PDB: 4HP9) complexed with the C-linker/CNBHD model from alignments to the structure of the EAGD–CNBHD complex from mouse (PDB: 4LLO). Full size image Structural and functional properties of CNBHD mutations Mutations were mapped onto a homology model of the C-linker/CNBHD (residues 666–749) described in the methods ( Fig. 4c ; Supplementary Fig. 1c,d ). Each monomer consists of a β-roll motif containing a short β-strand, with F860 and L862 forming an ‘intrinsic ligand’ rather than a modulatory ligand (PDB: 3UKN) [19] , [35] , [53] . While the different trafficking-deficient phenotypes are scattered, showing no correlation with location, most of the uncorrectable mutations (red) lie inside the β-roll and near the intrinsic ligand, suggesting that disruption of this subdomain is highly destabilizing. ( Fig. 4c,d ). Previous studies have shown that a hydrophobic patch that interfaces with the EAGD, and an acidic patch are important for regulating Kv11.1 deactivation [30] , [36] ( Fig. 4d ; Supplementary Fig. 1e–h ). Surprisingly, of the trafficking-competent mutations, only R791W lies close to a gating microdomain at the interface with the EAGD. S706C, I711V and R835W are largely buried but near the C-linker/CNBHD dimer interface, while D767Y is not located near any known gating microdomain ( Supplementary Fig. 1c,g,h ). To determine their electrophysiological properties, stable cell lines were generated for each of these with representative immunoblots and I Kv11.1 densities as shown in Supplementary Fig. 2A . The functional properties of S706C were similar to those of WT, in contrast to a previous report showing small changes in gating ( Table 1 ; Fig. 3e–h ) [36] . The V 1/2 of D767Y and R791W were both shifted by −12 mV, while that for R835W was shifted by +16 mV ( Fig. 3e,f ), and deactivation measured at −50 mV for I711V, R791W and R835W was faster compared to WT ( Fig. 3g ). To our knowledge, these are the first reports of class 3 (altered gating) LQT2-linked CNBHD mutations studied in a mammalian expression system. Trafficking of homomeric pore mutations At least 100 pore missense mutations have been linked to LQT2, yet the majority remain uncharacterized. To determine their trafficking phenotype, we used the same immunoblot assay and colour-code presentation described for the EAGD with the exception of orange indicating E4031 correctable only. 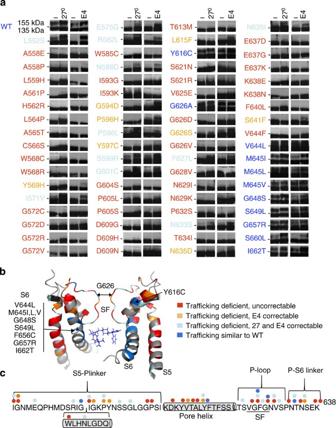Figure 5: Trafficking phenotype of LQT2-linked pore missense mutations. (a) Representative immunoblots of transiently transfected HEK293 cells comparing trafficking under control conditions at 37 °C, at reduced temperature (27 °C) or in E4031 (E4). Dashes (−) indicate the 140-kDa molecular weight marker. Mutations are colour-coded as follows: trafficking deficient and uncorrectable in red, trafficking deficient but correctable at 27 °C or with E4031 in light blue, trafficking deficient but only correctable with E4031 in orange, and those that traffic similar to WT in blue. (b) Structural model of the pore with Terfenadine (blue molecule) modelled into the putative drug-binding domain54. Mapped LQT2 residues correspond to panelaand uncharacterized mutations (M574R and L622F) are in black. (c) Linear representation of the S5–S6 pore linker with helices represented as cylinders and coloured dots representing the different trafficking phenotypes associated with each residue (for example, G626). Figure 5a shows representative immunoblots ( n ≧ 2) for 71 mutations. In all 60 (85%) lacked a 155-kDa band on immunoblot compared to WT under control culture conditions. Of these, 12 (20%) were correctable with culture at 27 °C and 20 (33%) were correctable with culture in E4031. Interestingly, eight were only E4031 correctable and none were only temperature correctable, in contrast to the PASD and CNBHD. These data, combined with several mutations already reported in the literature, are summarized in Supplementary Table 4 . Figure 5: Trafficking phenotype of LQT2-linked pore missense mutations. ( a ) Representative immunoblots of transiently transfected HEK293 cells comparing trafficking under control conditions at 37 °C, at reduced temperature (27 °C) or in E4031 (E4). Dashes (−) indicate the 140-kDa molecular weight marker. Mutations are colour-coded as follows: trafficking deficient and uncorrectable in red, trafficking deficient but correctable at 27 °C or with E4031 in light blue, trafficking deficient but only correctable with E4031 in orange, and those that traffic similar to WT in blue. ( b ) Structural model of the pore with Terfenadine (blue molecule) modelled into the putative drug-binding domain [54] . Mapped LQT2 residues correspond to panel a and uncharacterized mutations (M574R and L622F) are in black. ( c ) Linear representation of the S5–S6 pore linker with helices represented as cylinders and coloured dots representing the different trafficking phenotypes associated with each residue (for example, G626). Full size image Structural and functional properties of pore mutations Mutations were mapped onto a previously published model of the open state ( Fig. 5b ) [54] . A few patterns emerge. First, most of the trafficking-competent mutations are located in S6. Second, most S5 mutations have a severe trafficking phenotype, with all 14 being trafficking deficient and only 2 correctable. Finally, most trafficking-deficient but correctable mutations lie in the pore linker between S5 and S6 ( Fig. 5b,c ). Similar to the PASD and C-linker/CNBHD, some residues contain more than one LQT2-linked mutation with different trafficking phenotypes ( Fig. 5c ). For example, G626A in the selectivity filter traffics normally, whereas G626D and G626V are trafficking deficient and uncorrectable and G626S is only E4031 correctable ( Fig. 5a,b ). To determine if the trafficking-competent pore mutations express currents, stably transfected cell lines were generated for V644L, S649L, G657R (a conserved glycine) and I662T, all located in S6, as well as Y616C located in the pore helix. All showed a 155-kDa band, but only V644L, G657R and I662T expressed large-amplitude I Kv11.1 ( Supplementary Fig. 2a ). By contrast, stable cell lines for Y616C (6.0±1.0 pA pF −1 , n =8) and S649L (2.5±0.6 pA pF −1 , n =8) showed minimal I Kv11,1 , suggesting a class 4 (altered permeation) mechanism. For the G657R mutation, depolarizing voltage steps to −70 to 50 mV also resulted in activation of no outward I Kv11,1 , whereas a low-amplitude inward tail current was elicited by a voltage step to −120 mV, suggesting a class 3 mechanism ( Supplementary Fig. 2b,c ). The functional properties of I662T were similar to WT, but V644L exhibited faster inactivation measured at 0 mV consistent with a class 3 (abnormal gating) mechanism ( Table 1 ; Fig. 6c–f ). 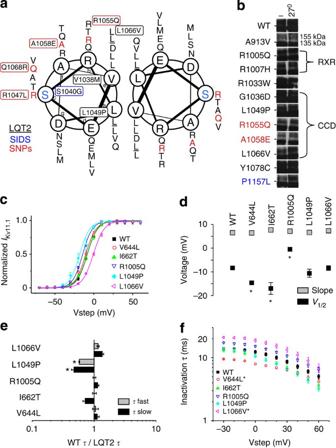Figure 6: Trafficking phenotype of LQT2-linked distal C-terminal missense mutations. (a) Helical wheel diagram showing two of the four helices forming the coiled-coil domain with LQT2 mutations underlined in black, SIDS mutations in blue and SNPs in red. (b) Representative immunoblots of transiently transfected HEK293 cells comparing trafficking under control conditions at 37 °C and at reduced temperature (27 °C). Dashes (−) indicate the 140-kDa molecular weight marker. (c)I–Vrelationships. (d)V1/2and slope factors. (e) WT-to-mutant time constant ratios (speeding factor) for deactivation at −50 mV. (f) Inactivation time constants determined at 0 mV. Protocols are described inFig. 3. Error bars are s.e.m. Asterisks indicate statistical significance (P≪0.05).n=4 to 12 HEK293 cells for each experiment. Figure 6: Trafficking phenotype of LQT2-linked distal C-terminal missense mutations. ( a ) Helical wheel diagram showing two of the four helices forming the coiled-coil domain with LQT2 mutations underlined in black, SIDS mutations in blue and SNPs in red. ( b ) Representative immunoblots of transiently transfected HEK293 cells comparing trafficking under control conditions at 37 °C and at reduced temperature (27 °C). Dashes (−) indicate the 140-kDa molecular weight marker. ( c ) I – V relationships. ( d ) V 1/2 and slope factors. ( e ) WT-to-mutant time constant ratios (speeding factor) for deactivation at −50 mV. ( f ) Inactivation time constants determined at 0 mV. Protocols are described in Fig. 3 . Error bars are s.e.m. Asterisks indicate statistical significance ( P ≪ 0.05). n =4 to 12 HEK293 cells for each experiment. Full size image Several LQT2-linked mutations introduce a polar residue or proline and may decrease membrane insertion efficiency, a mechanism underlying other membrane protein-misfolding diseases [55] , [56] , [57] . Using the ΔG predictor tool [58] , we found that 10 of 17 S5 mutations, but only 1 in S6, are predicted to insert less efficiently (ΔΔG ≧ 0.5), which might partially explain why most S5 mutations have a severe trafficking phenotype that is not correctable and most in S6 mutations traffic normally. Mutations in S1–S4 were also modeled using the ΔG predictor tool and only 2 of 20 mutations (both in S1) had a ΔΔ G ≧ 0.5. Interestingly, several mutations in S2 and S3 and all in S4 occur at charged residues important for voltage sensing, but these also may be important for membrane insertion ( Supplementary Table 5 ) [59] . Structural and functional properties of C-terminal mutations The distal C-terminus (residues beyond the CNBHD) contains at least 36 (31 LQT2, 5 SIDS) mostly uncharacterized mutations and 16 SNPs, several of which are located in or near the CCD and ER retention signal (RXR) ( Figs 1a and 6a ). Immunoblot analysis ( n ≧ 2) of transiently transfected HEK293 cells revealed that all eight LQT2 mutations, one SIDS and two SNPs tested traffic similar to WT ( Fig. 6b ). To determine their electrophysiological properties, stably transfected HEK293 cells were generated for R1005Q in the RXR as well as L1049P and L1066V, which are at the hydrophobic interface of the CCD ( Supplementary Fig. 2a ). The V 1/2 of R1005Q and L1049P shifted −6 and −9 mV, respectively, and L1066V shifted +8 mV. L1049P also exhibited slower deactivation at −50 mV and L1066V exhibited slower inactivation at 0 mV ( Table 1 ; Fig. 7c–f ). Interestingly, Paircoil2 analysis predicted that L1049P, but not L1066V, disrupts the CCD, which might explain their slightly different functional characteristics even though they are similarly located. 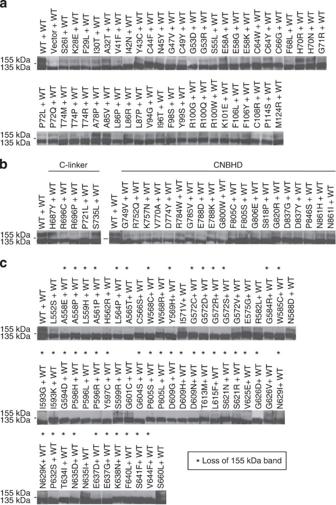Figure 7: Trafficking phenotype of LQT2 missense mutations co-expressed with WT. Representative immunoblots of transiently transfected HEK293 cells co-expressing WT with (a) PASD mutants, (b) C-linker/CNBHD mutants, or (c) pore mutants as heteromeric channels under control conditions. Dashes (−) indicate the 140-kDa molecular weight marker. Asterisks (*) indicate complete absence of the 155-kDa band. Figure 7: Trafficking phenotype of LQT2 missense mutations co-expressed with WT. Representative immunoblots of transiently transfected HEK293 cells co-expressing WT with ( a ) PASD mutants, ( b ) C-linker/CNBHD mutants, or ( c ) pore mutants as heteromeric channels under control conditions. Dashes (−) indicate the 140-kDa molecular weight marker. Asterisks (*) indicate complete absence of the 155-kDa band. Full size image Trafficking of LQT2 mutations co-expressed with WT Since LQT2 is an autosomal dominant disease where only one abnormal allele is present, immunoblots were also performed on HEK293 cells co-transfected with equal amounts of WT and mutant DNA. Immunoblot analysis ( n ≧ 2) showed that nearly all missense mutants exhibited a diminished 155-kDa band compared to WT alone ( Fig. 7a–c ). A few mutations such as H70R and A78P in the PASD, H687Y and S735L in the CNBD, and S660L in the pore showed a 155-kDa band similar to WT. However, in contrast to the PASD and CNBHD, where nearly every mutation showed at least a weak 155-kDa band, 44 of 58 (76%) pore mutations completely lacked a 155-kDa band ( Fig. 8c , indicated as *). Thus, in the pore domain the presence of mutant α-subunit(s) is strictly dominant-negative for the majority of mutations. 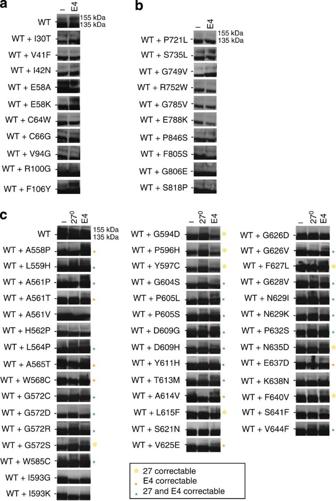Figure 8: Correction of heteromeric Kv11.1 channels. Representative immunoblots of transiently transfected HEK293 cells co-expressing WT with (a) PASD mutants, (b) C-linker/CNBHD mutants, or (c) pore mutants as heteromeric channels under control conditions (−), with culture at 27 °C (24 h) or culture in E4031 (E4, 24 h). Dashes (−) indicate the 140-kDa molecular weight marker. Yellow, orange and blue asterisks indicate correction at 27 °C, in E4031 or both, respectively, that were not correctable under those conditions as homomeric channels. H562P is also included, which was not completely dominant negative. Figure 8: Correction of heteromeric Kv11.1 channels. Representative immunoblots of transiently transfected HEK293 cells co-expressing WT with ( a ) PASD mutants, ( b ) C-linker/CNBHD mutants, or ( c ) pore mutants as heteromeric channels under control conditions (−), with culture at 27 °C (24 h) or culture in E4031 (E4, 24 h). Dashes (−) indicate the 140-kDa molecular weight marker. Yellow, orange and blue asterisks indicate correction at 27 °C, in E4031 or both, respectively, that were not correctable under those conditions as homomeric channels. H562P is also included, which was not completely dominant negative. Full size image To determine if co-expression of mutant+WT alleles changes the trafficking phenotype of HEK293 cells cultured in E4031, immunoblot analysis ( n ≧ 2) was performed on 10 PASD mutations and no differences were found from homomeric channels. Eight mutations remained uncorrectable with culture in E4031, while two positive controls (F106Y and E58K) were still correctable ( Fig. 8a ). Similarly, co-expression of WT+10 C-linker/CNBHD mutations was tested and no differences in E4031 response were found ( Fig. 8b ). However, when 42 pore mutations were co-expressed with WT, including four previously reported (A561P, A561T, Y611H and A614V) [10] , 35 (83%) showed enhancement of the 155-kDa band ( Fig. 8c ). Of these 35, 20 demonstrated improvement of the 155-kDa band with culture at reduced temperature or with E4031 that was not correctable with reduced temperature or with E4031 as homomeric channel (blue asterisks). Seven showed improved trafficking with E4031 that was not correctable with E4031 as homomeric channel (orange asterisks), and 8 could be corrected with reduced temperature that was not temperature correctable as homomeric channels (yellow asterisks). Thus, in the pore domain, correction of trafficking-deficient mutations depends on α-subunit composition and is enhanced by the addition of WT α-subunits. Our data-driven approach provides new insights into LQT2 that would not have otherwise been possible. First we identified a loss-of-function mechanism for most of the LQT2-linked missense mutations in three structural domains. Including previously published findings with our present findings ( Fig. 9b and Supplementary Tables 1–4 ), 193 PASD, C-linker/CNBHD and pore mutations have been studied and 169 (88%) demonstrate a class 2 (trafficking-deficient) mechanism. This is in contrast to a smaller study of 10 PASD mutations that suggested most traffic normally [28] , underscoring the importance of this comprehensive large-scale analysis. Of the mutations studied electrophysiologically, nine show evidence for being class 3 (abnormal gating), including several shown for the first time in the CNBHD. Four were trafficking competent and generated minimal or no current, suggesting either a severe class 3 or a class 4 (altered permeation) mechanism. Several ‘mutations’ behave similar to WT, including most in the distal C-terminus, and it is unclear whether they are true LQT2 disease-causing mutations or benign variants. 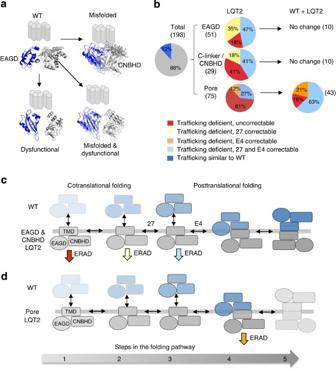Figure 9: Model of Kv11.1 biogenesis and correction. (a) Model illustrating class 2 and/or class 3 loss-of-function phenotypes for EAGD and C-linker/CNBHD mutations. Mutations can either be destabilizing, resulting in misfolding and ERAD (top right, out of focus), or disrupt protein–protein interactions, resulting in quicker deactivation (bottom left, separated) or both (bottom right). (b) Summary of the trafficking phenotypes by domain for Kv11.1 homomeric channels and channels co-expressed with WT. Number of mutations analysed are in parentheses (see alsoSupplementary Tables 2–4). (c,d) Simplified five-step folding model illustrating the different correction phenotypes based on the data reported here and elsewhere (see Discussion). (c) The most destabilizing EAGD and C-linker/CNBHD mutations fail to make it to step 2 and undergo ERAD (red). These are uncorrectable at 27 °C or with E4. Less destabilizing mutations make it further along the folding pathway (step 2) and are amenable to 27 °C temperature correction but not E4 pharmacological correction (yellow). Mildly destabilizing mutations make it to step 3, where E4031, which acts posttranslationally, can facilitate cooperative interactions between subunits, allowing for correction13. (d) Pore mutations (orange) behave differently. Most are stable enough to make it to step 4, but result in severe dominant-negative effects causing both WT and mutant to undergo ERAD. These heteromeric channels fail to make it to step 5 (dashed outlines) required for ER exit, but can undergo improved folding and ER exit with pharmacological correction strategies. Figure 9: Model of Kv11.1 biogenesis and correction. ( a ) Model illustrating class 2 and/or class 3 loss-of-function phenotypes for EAGD and C-linker/CNBHD mutations. Mutations can either be destabilizing, resulting in misfolding and ERAD (top right, out of focus), or disrupt protein–protein interactions, resulting in quicker deactivation (bottom left, separated) or both (bottom right). ( b ) Summary of the trafficking phenotypes by domain for Kv11.1 homomeric channels and channels co-expressed with WT. Number of mutations analysed are in parentheses (see also Supplementary Tables 2–4 ). ( c , d ) Simplified five-step folding model illustrating the different correction phenotypes based on the data reported here and elsewhere (see Discussion). ( c ) The most destabilizing EAGD and C-linker/CNBHD mutations fail to make it to step 2 and undergo ERAD (red). These are uncorrectable at 27 °C or with E4. Less destabilizing mutations make it further along the folding pathway (step 2) and are amenable to 27 °C temperature correction but not E4 pharmacological correction (yellow). Mildly destabilizing mutations make it to step 3, where E4031, which acts posttranslationally, can facilitate cooperative interactions between subunits, allowing for correction [13] . ( d ) Pore mutations (orange) behave differently. Most are stable enough to make it to step 4, but result in severe dominant-negative effects causing both WT and mutant to undergo ERAD. These heteromeric channels fail to make it to step 5 (dashed outlines) required for ER exit, but can undergo improved folding and ER exit with pharmacological correction strategies. Full size image Not surprisingly, we found that C-linker/CNBHD mutations behave similarly to PASD mutations. Since class 3 (abnormal gating) PASD mutations have been shown to disrupt ‘core’ interactions with the CNBHD [60] , class 3 CNBHD mutations likely act similarly. Indeed, to our knowledge we identified the first class 3 CNBHD mutations as well as the first class 2 (trafficking-deficient) CNBHD mutations that can be corrected with culture in E4031. Figure 9a illustrates these similarities, where most mutations are destabilizing, resulting in misfolded channels with reduced I Kv11.1 density but nearly normal gating (for example, G53R, H70R and A78P) [50] . Other mutations traffic normally but are located near gating microdomains, resulting in dysfunctional channels but with nearly normal I Kv11.1 density (for example, R56Q, N33T, R835W, R791W) [16] . Finally, other mutations are both destabilizing (misfolded) and located in gating microdomains (dysfunctional) (for example, K28E, F29L, M124R, R784W and E788K) [36] , [51] . This model might also help explain why G53R, H70R, A78P all exhibit faster deactivation in Xenopus oocytes but not in HEK293 cells [50] , [51] . Misfolding mutations lying outside gating microdomains will still fail to form the ‘core’ interactions necessary for proper function, but are not marked for degradation in Xenopus oocytes, which are cultured at reduced temperature. However, the opposite is true for S706C, which was reported to have faster deactivation in Xenopus oocytes but not in this study using HEK293 cells [36] . Clearly, differences between expression models need to be considered when evaluating LQT2 mutations, and perhaps studies in more native model systems would be useful [61] , [62] . Several lines of evidence suggest that correction of trafficking-deficient intracellular PASD and CNBHD mutations works at different steps along the folding pathway as illustrated in Fig. 9c . This model is supported by the following observations: (1) correction strategies typically work only for missense mutations with a diminished 155-kDa band, but not for mutations completely lacking a 155-kDa band; (2) the trafficking phenotype for several PASD mutations has been shown to correlate with domain stability [28] , [63] ; (3) all PASD and C-linker/CNBHD mutations that are E4031 correctable are also temperature correctable, suggesting that E4031 works further along the folding pathway where the pore is intact; and (4) E4031 acts posttranslationally [13] . Since the majority of mutations are correctable and therefore likely only slightly destabilizing, strategies that improve domain stability could help many LQT2–Kv11.1 channels evade ERAD [64] . Pore mutations are strikingly different from intracellular domain mutations. Two-thirds act in a completely dominant-negative manner when co-expressed with WT, in contrast to intracellular mutations ( Fig. 9d ). Furthermore, heteromeric channels are much more amenable to pharmacological correction than homomeric channels ( Fig. 9b ). These results provide an explanation for the increased clinical severity of pore mutations, but also show more promise for pharmacological chaperones as a possible therapeutic approach [65] . While these studies have provided several new molecular insights into LQT2, many important questions remain. Since co-expression of WT can improve mutant Kv11.1 channel dysfunction [66] , functional studies of co-expressed channels are needed. For example, Kv11.1 G657R appears to behave similar to a Shaker channel mutation that converts it from a K + channel passing outward current to a K + channel passing inward current at negative voltages [67] . What loss-of-function mechanisms, if any, underlie the other Kv11.1 structural regions like the VSD [68] or the linker regions? Interestingly, as shown in Fig. 1 , all reported SNPs lie in linker regions of the Kv11.1 protein lacking a highly ordered structure except for the CCD; thus, these areas may be more tolerant of amino-acid substitutions. Using the sequence-based prediction tools SIFT, SNP&Go and KvSNP, only 21–73% of mutations and 11–46% of SNPs were predicted to be pathogenic compared to 80–99% in structural domains (see Supplementary Tables 1 and 6 ). What are the structural bases for Kv11.1 misfolding? This is a largely unexplored area, but especially important since LQT2 is predominantly a misfolding disease. For example, do LQT2 missense mutations disrupt intra (local) and/or interdomain (global) interactions [69] ? Do TMD mutations insert less efficiently as predicted, which has been demonstrated for other channelopathies [55] , [56] ? Does L1049P disrupt the CCD as predicted? As a final example, it was surprising that both LQT2 mutations in the ER retention signal (R1005Q and R1007H) traffic normally. This suggests that these mutations do not disrupt binding of the distal C-terminus, which is thought to mask the RXR signal [20] . These questions and many others remain unresolved, but this large-scale mutational analysis has shed new light on LQT2 disease mechanisms and may help the efforts towards developing rational approaches to predicting the pathogenic mechanism(s) of newly discovered Kv11.1 variants and correction strategies as clinically useful therapeutic options [70] . Mutation database and mutagenesis LQT2-associated Kv11.1 missense mutations were identified predominantly from the Inherited Arrhythmias Database ( www.fsm.it/cardmoc ) and published genotyping from the various literature sources listed in Supplementary Table 1 . All missense mutations were made using the QuikChange II XL kit from Agilent (Santa Clara, CA) using primers designed with their primer design program and obtained from Integrated DNA Technologies (Coralville, IA). A pcDNA3 WT HERG1a expression construct previously published was used as the template [10] . Restriction digest analysis was used to test the integrity of all constructs and all mutations were verified by sequencing at the UW-Biotechnology Center. Bioinformatics PASD structural models were created in Pymol using PDB: 1BYW. A Clinker/CNBHD structural model (Kv11.1 amino acids 672–864) was generated by Swiss-Model using the C-terminal structure from the homologous zELK KCNH (PDB: 3UKN) as a template. The quality of the model was evaluated using Molprobity and scored in the 56th percentile (100% being the best). After energy minimization using UCSF Chimera’s minimization function, the model improved to the 91st percentile and was used for all subsequent modelling. Mutation pathogenicity was also evaluated for all mutations using the sequence-based programs SIFT, KvSNP, and SNPs&Go. Membrane insertion efficiency was predicted using the ΔG predictor. This tool predicts the apparent free energy difference for membrane insertion based on an experimentally determined biological hydrophobicity scale. Paircoil 2 was used to predict coiled-coil formation. Web servers and literature sources are listed in Supplementary Table 7 . Kv11.1 trafficking HEK293 cells of similar confluence were transiently transfected with SuperFect (Qiagen) and grown at 37 °C for 24 h before study. Transfections were done with 3 μg of cDNA for homomeric expression or 1.5 μg mutant +1.5 μg WT cDNA for co-expression. To test for correction of deficient Kv11.1 protein trafficking, cells were grown for an additional 24 h at 37 °C for control, or at 27 °C, or in the presence of 10 μM E4031 (Alamone). Immature and mature Kv11.1 protein bands were detected by immunoblot analysis of whole-cell lysates. Briefly, lysates were mixed with an equal amount of Laemili sample buffer, separated by 7% SDS-PAGE, and transferred to a nitrocellulose paper. Blots were incubated with a rabbit antibody (1:10,000) directed to the distal C-terminus as previously described [9] , [10] . Bands were detected with a goat anti-rabbit secondary antibody conjugated to HRP. Uncropped western blots are shown in Supplementary Fig. 2e . Kv11.1 function Stable cell lines were generated by transfecting HEK293 cells with mutant HERG pcDNA3 and selecting in G418 as previously described [10] . Single colonies of G418-resistant cells were then tested for Kv11.1 expression by immunoblot. Cell lines that gave a robust 155-kDa band on immunoblot were used for electrophysiological analysis. I Kv11.1 was measured using the whole-cell patch clamp technique as previously described [10] . Voltage protocols are described in the Fig. 3 legend and data analysis was done using pCLAMP 8.0 (Axon Instruments) and Origin (6.0 Microcal). Statistical analysis All data are presented as mean±s.e. One-way analysis of variance (ANOVA) was used for statistical analysis followed by the Tukey post hoc test. P ≪ 0.05 was considered statistically significant. How to cite this article: Anderson, C. L. et al. Large-scale mutational analysis of Kv11.1 reveals molecular insights into type 2 long QT syndrome. Nat. Commun. 5:5535 doi: 10.1038/ncomms6535 (2014).